In vivoformation of double-stranded T-DNA molecules by T-strand priming During plant genetic transformation, Agrobacterium transfers a single-stranded DNA (T-strand) into the host cell. Increasing evidence suggests that double-stranded (ds) T-DNA, converted from T-strands, are potent substrates for integration. Nevertheless, the molecular mechanism governing T-strand conversion to dsT-DNA is unknown. Integrated T-DNA molecules typically exhibit deletions at their 3′ end as compared with their 5′ end. We hypothesize that this may result from asymmetric polymerization of T-DNA’s ends. Here we show that β-glucuronidase (GUS) expression from sense T-strands is more efficient than from antisense T-strands, supporting asymmetric conversion. Co-transfection with two partially complementary, truncated GUS-encoding T-strands results in GUS expression, which suggests functional hybridization of the T-strands via complementary annealing and supports the notion that T-strands can anneal with primers. Indeed, red fluorescent protein (RFP) expression from mutated T-strand can be restored by delivery of synthetic DNA and RNA oligonucleotides with partial wild-type RFP sequence, implying the involvement of plant DNA repair machinery. A grobacterium genetically transforms its host by delivering its transferred DNA (T-DNA) into the host genome, where it is stably integrated and expressed. The T-DNA, defined by two 25-bp direct-repeat border sequences, travels as a single-stranded (ss) DNA molecule (T-strand), with a single Agrobacterium VirD2 protein attached to its 5′ end [1] , [2] , [3] . Once inside the plant cell, the VirD2-capped T-strand is thought to be packed by numerous Agrobacterium VirE2 proteins [4] , [5] . Both VirD2 and VirE2 are thought to function during T-strand nuclear import and intra-nuclear transport [6] , [7] , [8] . VirD2 may also function during the genomic integration of the T-DNA through unknown mechanisms [9] , [10] . The T-DNA sequence does not code for the machinery needed for its transport or integration into the plant genome and it can therefore be replaced by virtually any other sequence without affecting the transformation process. T-DNA molecules integrate at random locations across the plant genome possibly via non-homologous end joining, and are only rarely directed to and integrated in specific genomic locations by homologous recombination [11] , [12] , [13] . Sequence analysis of integration events has revealed that integrated T-DNAs often lose part of their 3′ end, while the 5′ end can remain intact [13] , [14] , [15] , [16] , [17] . Various models have been proposed to explain the structure of integration events and the random nature of T-DNA integration into the plant genome; of these, the microhomology-based T-DNA integration models are predominant [10] , [18] . According to these models, integration is initiated by annealing of the 3′ or 5′ end of the T-strand to unwound plant DNA at pre-integration genomic sites, followed by nicking of the target DNA, ligation of the 5′ end to one of the target DNA strands and trimming of the T-strand’s unprotected 3′ end [10] , [18] . Alternatively, the T-strand might be converted into double-stranded (ds) T-DNA molecules in the plant cell, which can then integrate into genomic double-strand breaks (DSBs) [11] , [19] , [20] . While the direct integration of T-strand molecules cannot be ruled out, the rapid and efficient conversion of T-strands to dsT-DNA suggests that the latter may serve as an important substrate for the integration machinery. Notably, dsT-DNA molecules are important substrates for many recombinase-mediated gene-replacement and site-specific-integration systems [21] , [22] . However, the mechanism by which T-strands are converted into dsT-DNAs is still unknown. Here we use several functional assays to investigate the process of T-strand conversion into dsT-DNA molecules. We show that the expression of the β-glucuronidase (GUS) encoding gene from sense T-strands is more efficient than from antisense molecules and that the co-transfection of tobacco leaves with two partially complementary, truncated GUS-encoding T-strands, but not with individual or partially overlapping truncated GUS-encoding T-strands, results in GUS expression. Using functional mutated red fluorescent protein (RFP)-repair assay, we demonstrate that T-strand molecules can anneal with nucleic acid primers in vivo . A model of dsT-DNA formation in plant cells is suggested. Detecting in vivo formation of dsT-DNAs by functional assay Given that the nature of T-strand conversion to a double-stranded form is a process of DNA polymerization, it may be initiated by T-strand priming by short plant primers. Such primers can be de-novo -synthesized RNA primers or endogenous pre-existing ssDNA or RNA fragments. Because priming may occur at random locations along the T-strand and DNA polymerization follows the 5′ to 3′ direction, the resulting dsT-DNA intermediates may remain single-stranded at the ends, and in particular at their 3′ ends. These single-stranded regions are susceptible to nuclease degradation, potentially leading to truncations of dsT-DNA molecules, in particular at their 3′ ends. Indeed, sequencing data of T-DNA integration sites have revealed that the 3′ end of a T-DNA is more vulnerable to deletion than its 5′ end [14] , [15] , [16] , [17] . We hypothesized that truncation of T-DNA ends (in particular at the 3′ end) may arise, at least partially, from incomplete T-strand to double-stranded conversion, which occurs before the integration step. Notably, truncation of T-DNA ends (especially the 3′ end) may also occur during T-DNA integration, as suggested by Tinland et al . [10] in their ssT-DNA integration model. We tested our hypothesis by monitoring the formation of dsT-DNA intermediates using a functional assay, in which transient expression of the GUS reporter gene occurs independently of T-DNA integration, in a manner similar to this assay’s previous use to determine that T-DNAs are transferred as single-stranded, but not double-stranded molecules into the plant cell nucleus [2] . In our assay, two binary vectors were engineered to produce either sense (S, Fig. 1a ) or antisense (AS, Fig. 1a ) T-strand molecules of the same functional GUS expression cassette. The structure of our GUS expression cassettes included a long 886-bp dual 35S CaMV promoter and a short 211-bp 35S CaMV terminator. In the design of our vectors, even moderate deletions at the 3′ end are likely to interfere with GUS expression in sense T-strand molecules because of the relatively short terminator region (~350 bp from the beginning of the terminator to the end of the T-DNA’s border region); however, because a single 35S CaMV promoter (and even just a minimal promoter sequence [23] ) is sufficient to produce GUS expression, larger deletions (that is, longer than 750 bp, in our constructs) at the 3′ end will be required to interfere with GUS expression in antisense T-strand molecules. This may lead to a difference in GUS expression between transfected sense and antisense T-strands. In fact, infection of tobacco leaves with an identical concentration of Agrobacterium cells carrying sense or antisense T-strand molecules showed that GUS expression from antisense T-strands is more efficient than from sense T-strands (compare AS with S, Fig. 1b ). This observation is compatible with the hypothesized 3′ deletion of pre-integrated T-DNA, implicating an alternative mechanism for the frequently observed 3′ truncation of integrated T-DNA. This possible mechanism emphasizes the notion that the double-stranded conversion stabilizes T-DNA by inhibiting nuclease degradation of its single-stranded form; whereas, the random annealing nature of the primers along the T-strand may not be able to initiate its complete conversion, leaving the non-complementary portion, more likely to be the 3′ end, susceptible to degradation. Note that aside from the possible asymmetrical double-stranded conversion of the 5′ and 3′ ends, other factors, such as suggested VirD2 protection of the 5′ end [24] , might also contribute to the unequal stability of these two ends. Interestingly, GUS expression in leaves which were co-infected with both sense and antisense Agrobacterium strains, each at half concentration, was more efficient than in leaves infected by individual strains at full concentration (compare S+AS with S or AS, Fig. 1b ). It has been shown that GUS expression can be restored by hybridization of two putative T-strand molecules [2] and we thus suggested that in these co-infection experiments, the sense and antisense T-strand molecules, which may have been stripped of their escorting VirE2 molecules [25] , [26] , hybridized with each other and produced an artificial dsT-DNA, most likely with higher efficiency and stability than the natural conversion of individual T-strands. 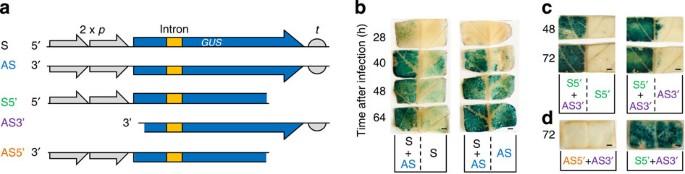Figure 1: Detection of T-strand conversion to dsT-DNA byin vivoannealing of complementary T-strands. (a) Schematic of several constructed T-strand molecules. S and AS molecules carry the sense or antisense strand of a functional GUS expression cassette, respectively. S5′, AS3′ and AS5′ molecules carry the sense (S5′) or antisense (AS3′ and AS5′) strand of two partial, non-functional, yet overlapping GUS expression cassettes, respectively. The GUS expression cassette contains an intron to prevent its expression inAgrobacterium. (b–d) Analysis of GUS expression in infected tobacco leaves at different time points afterAgrobacteriuminfiltration. TheAgrobacteriumstrains used for the infiltration are indicated in each sample. Bars are 2 mm in length. 2 xp, dual 35S promoter;t, 35S terminator;GUS, β-glucuronidase-encoding gene. Figure 1: Detection of T-strand conversion to dsT-DNA by in vivo annealing of complementary T-strands. ( a ) Schematic of several constructed T-strand molecules. S and AS molecules carry the sense or antisense strand of a functional GUS expression cassette, respectively. S5′, AS3′ and AS5′ molecules carry the sense (S5′) or antisense (AS3′ and AS5′) strand of two partial, non-functional, yet overlapping GUS expression cassettes, respectively. The GUS expression cassette contains an intron to prevent its expression in Agrobacterium . ( b – d ) Analysis of GUS expression in infected tobacco leaves at different time points after Agrobacterium infiltration. The Agrobacterium strains used for the infiltration are indicated in each sample. Bars are 2 mm in length. 2 x p , dual 35S promoter; t , 35S terminator; GUS , β-glucuronidase-encoding gene. Full size image In vivo hybridization of single-stranded T-DNAs In vivo annealing of two partially complementary T-strands or a single T-strand carrying inverted repeats was reported, in support of the notion that T-DNA is transferred in single-stranded form from Agrobacterium to its host [2] . We thus took advantage of such T-strand annealing to unequivocally test whether annealed T-strands can serve as primers (and by implication as DNA and RNA oligonucleotides) to initiate the formation of dsT-DNA. Note that in our design (S5′ and AS3′, Fig. 1a ), we intentionally infected cells with two T-strands, each with polymerase-extendable 3′ ends. This design allowed us to investigate the elongation of the priming T-strand by plant DNA polymerases using the annealed T-strand as template. We infected tobacco leaves with T-DNA molecules, which were engineered to carry non-functional portions of the GUS expression cassette (S5′ and AS3′, Fig. 1a ). As expected, no GUS expression was observed in these leaf samples (S5′ and AS3′, Fig. 1c ). However, GUS expression was clearly observed in leaf samples co-infected with two independent Agrobacterium strains, each carrying a different truncated T-DNA molecule (compare the combination of S5′+AS3′ with S5′ or AS3′, Fig. 1c ). The restoration of GUS expression was likely caused by in vivo annealing and subsequent DNA polymerization of two truncated T-strands. Alternatively, it might have derived from homologous recombination between dsS5′ and dsAS3′ intermediates. To rule out the latter possibility, we produced an antisense version of S5′, designated AS5′ ( Fig. 1a ), in which a truncated S5′ molecule was delivered in an antisense orientation, and we used it in co-infection experiments with AS3′ ( Fig. 1a ). Figure 1d shows that although clear GUS expression was observed in leaf samples co-infected with strains S5′ and AS3′, no GUS expression was observed in leaf samples co-infected with strains AS5′ and AS3′. These observations clearly support the notion that the detected reconstitution of a functional GUS-expressing T-DNA from truncated T-strand molecules is derived from annealing of the sense and antisense T-strands and not from recombination between two homologous dsT-DNA molecules. Importantly, they also suggest that the 3′ end of a complementary ssDNA fragment can serve as an initiation point for DNA polymerization, using the primary strand (that is, T-strand) as template. Note that while we did not detect homologous recombination between dsS5′ and dsAS3′ intermediates, we cannot exclude the occurrence, albeit at low frequency, of such events. T-strand-repair assay unveils priming of T-strand molecules To further investigate the notion that short nucleic acid fragments are capable of priming T-strands, and the function of these fragments as initiation points for polymerization of the nascent strand, we developed a T-strand-repair assay which allowed monitoring of the annealing and elongation of an artificial T-strand primer (cRFP, Fig. 2a,b ) and at least one more, endogenous, plant primer on the target T-strand (T-RFP, Fig. 2a,b ). The T-strand molecule, T-RFP, was engineered to carry two independent and functional constitutive plant expression cassettes. The first cassette, which was cloned near the T-DNA’s right border, expressed the EYFP protein tagged with endoplasmic reticulum (ER)-bound chalcone synthase (CHS), while the second cassette expressed the RFP protein tagged with nuclear localization signal (NLS). We used confocal fluorescence microscopy to monitor T-strand conversion to dsT-DNA in Agrobacterium -infected tobacco leaves. As expected, T-RFP-infected cells exhibited both ER-bound EYFP and nuclear RFP signals (T-RFP, Fig. 3 ). We next produced two mutated variants of T-RFP, designated T-mutRFP-1 and T-mutRFP-2, in which the RFP-coding sequence was interrupted with a 1 or 11-nt long insertion, respectively ( Fig. 2b ). As expected, these mutations interfered with RFP, but not with EYFP expression in infected leaves (T-mutRFP-1 and T-mutRFP-2, Fig. 3 ). We also constructed a T-strand molecule, cRFP ( Fig. 2a,b ), which was engineered to carry a partial wild-type RFP sequence (~500 nt long) that is complementary to the mutated RFP region of T-mutRFP-1 and T-mutRFP-2. An antisense version of the cRFP molecule, anti-cRFP, was also constructed ( Fig. 2b ). Annealing of cRFP to T-mutRFP-1 and T-mutRFP-2 creates a bulging or mismatched DNA region [27] , of which DNA repair may restore the wild-type RFP -coding sequence in T-mutRFP-1 and T-mutRFP-2 if cRFP was recognized as the repair template. Co-transformation of T-mutRFP-1 or T-mutRFP-2 with cRFP resulted in restoration of RFP expression in some of the infected cells ( Fig. 3 ). However, RFP expression was not restored when T-mutRFP-1 was co-transformed with anti-cRFP ( Fig. 3 ). These observations indicated that restoration of RFP expression is derived from annealing between complementary T-strand molecules (for example, between T-mutRFP-1 and cRFP) but not by putative recombination between homologous dsT-DNA intermediates. Note that in addition to the short wild-type RFP sequence, cRFP also carries parts of the binary vector sequence (~100 nt long) on both ends, including the remaining border sequence and the junction sequence between the border and the RFP sequence ( Fig. 2a ). Therefore, restoration of RFP expression could only occur if the cRFP molecule’s left and right border tails had been trimmed and the DNA bulge between cRFP and T-mutRFP-1 or T-mutRFP-2 had been repaired. Efficient restoration of RFP expression in our assay strongly suggested that T-strand hybrids were substrates for the plant DNA repair machinery, thus supporting the notion that plant DNA repair machinery is actively involved in T-strand to dsT-DNA conversion. Finally, because the restoration of RFP–NLS expression also depended on the complete double-stranded conversion of the RFP expression cassette, our data indicate that at least one other endogenous plant primer must have annealed to the 3′ end region of the T-mutRFP-1 and T-mutRFP-2 ( Fig. 2a ), initiating another continuous T-strand double-stranded conversion upstream of the cRFP annealing region. Our data also implicate the possible involvement of plant DNA ligase(s) in ligating the gaps of newly synthesized DNA fragments, similar to ligation of Okazaki fragments in lagging-strand DNA synthesis, forming consecutive dsT-DNA molecules. 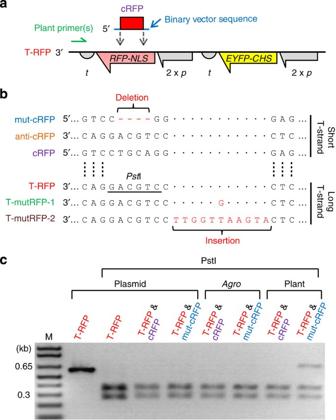Figure 2: Detection of T-strand conversion to dsT-DNA by site-specific mutagenesis. (a) Schematic ofin vivoannealing of T-RFP and cRFP molecules. Putative endogenous primer(s) (that is, plant primers) to initiate the double-stranded conversion of T-RFP’s 3′ end are presented. (b) Partial sequences of several T-strand constructs in theRFPregion bearing site-specific mutagenesis. T-RFP carries functional RFP–NLS and EYFP–CHS expression cassettes. T-mutRFP-1 and T-mutRFP-2 molecules carry a 1- or 11-nt insertion as indicated in the RFP-encoding sequence, respectively. cRFP carries a partial RFP-encoding sequence. Anti-cRFP is the complementary version of cRFP. mut-cRFP carries the same sequence as cRFP except for a 4-nt deletion in thePstI site, as indicated. cRFP, anti-cRFP and mut-cRFP serve as short T-strands, which can potentially anneal with long T-strands in the plant nucleus. (c) PstI digestion analysis of PCR products from T-RFP-specific PCR amplification. Extracted total DNA fromAgrobacterium-infected plant tissues and correspondingAgrobacteriumstrains and binary vector plasmids was used as templates for individual PCRs. 2 xp, dual 35S promoter;t, 35S terminator; M, DNA ladder. Figure 2: Detection of T-strand conversion to dsT-DNA by site-specific mutagenesis. ( a ) Schematic of in vivo annealing of T-RFP and cRFP molecules. Putative endogenous primer(s) (that is, plant primers) to initiate the double-stranded conversion of T-RFP’s 3′ end are presented. ( b ) Partial sequences of several T-strand constructs in the RFP region bearing site-specific mutagenesis. T-RFP carries functional RFP–NLS and EYFP–CHS expression cassettes. T-mutRFP-1 and T-mutRFP-2 molecules carry a 1- or 11-nt insertion as indicated in the RFP-encoding sequence, respectively. cRFP carries a partial RFP-encoding sequence. Anti-cRFP is the complementary version of cRFP. mut-cRFP carries the same sequence as cRFP except for a 4-nt deletion in the Pst I site, as indicated. cRFP, anti-cRFP and mut-cRFP serve as short T-strands, which can potentially anneal with long T-strands in the plant nucleus. ( c ) PstI digestion analysis of PCR products from T-RFP-specific PCR amplification. Extracted total DNA from Agrobacterium -infected plant tissues and corresponding Agrobacterium strains and binary vector plasmids was used as templates for individual PCRs. 2 x p , dual 35S promoter; t , 35S terminator; M, DNA ladder. 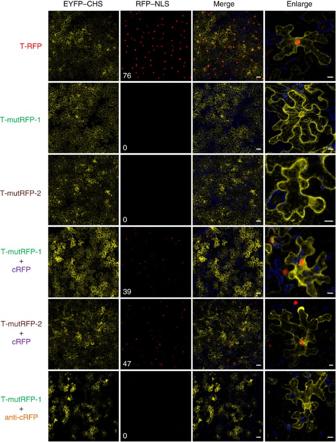Figure 3: Confocal fluorescence microscopy analysis ofin vivoformation of dsT-DNAs. Agrobacteriumstrains used for each infiltration are indicated on the left. From left to right: EYFP (yellow), RFP (red), merged image of EYFP, RFP and chlorophyll (dark blue) signals and enlargement of representative cell. Number of RFP–NLS-expressing cells is shown in the bottom left corner of each RFP–NLS image. Scale bars of merged images are 50 μm in length. Scale bars of enlarged images are 10 μm in length. Full size image Figure 3: Confocal fluorescence microscopy analysis of in vivo formation of dsT-DNAs. Agrobacterium strains used for each infiltration are indicated on the left. From left to right: EYFP (yellow), RFP (red), merged image of EYFP, RFP and chlorophyll (dark blue) signals and enlargement of representative cell. Number of RFP–NLS-expressing cells is shown in the bottom left corner of each RFP–NLS image. Scale bars of merged images are 50 μm in length. Scale bars of enlarged images are 10 μm in length. Full size image To confirm that DNA repair had indeed occurred in the bulging DNA region between the two T-strands, we engineered a mut-cRFP T-strand molecule carrying a 4-nt deletion which, on annealing to T-RFP, abolishes the Pst I site on the wild-type RFP-coding sequence ( Fig. 2b ). To detect the mutation by DNA repair, we designed a pair of primers that anneal to the RFP sequence surrounding, but outside of, the cRFP or mut-cRFP carrying sequence and are thus only able to amplify T-RFP, but not cRFP or mut-cRFP T-DNAs. Using this pair of primers, PCR amplification of mixtures of T-RFP with cRFP or mut-cRFP binary plasmids, as well as mixtures of Agrobacterium strains carrying T-RFP and cRFP or mut-cRFP binary plasmids, resulted in PstI-digestible products ( Fig. 2c ). In addition, PCR amplification of plants co-infected with T-RFP and cRFP resulted in PstI-digestible products ( Fig. 2c ). However, PCR amplification of plants co-infected with T-RFP and mut-cRFP yielded a PstI-indigestible band, which was similar in length to the undigested T-RFP PCR product ( Fig. 2c ). Sequencing analysis of the DNA recovered from this band confirmed the bona fide deletion in the PstI site. We should note that PstI-indigestible PCR products could have been amplified from either integrated or non-integrated T-DNAs. Given the relative amounts of PstI-indigestible and PstI-digestible products in the lane (plant: RFP and mut-cRFP), it is likely that most, if not all, of the PstI-indigestible product stemmed from non-integrated T-DNAs. In vivo priming of T-strand molecules by synthetic primers To further substantiate our hypothesis that DNA polymerization of the nascent strand is initiated by priming of short DNA and RNA fragments, we mimicked the putative natural process of T-strand conversion by testing whether short DNA and RNA oligonucleotides can serve as primers for this conversion. We used our T-strand-repair assay ( Fig. 2a ), except that this time we supplied T-strand-transformed cells with short complementary DNA or RNA oligonucleotides rather than a second T-strand molecule. We first infected tobacco leaves with Agrobacterium strain T-mutRFP-1 ( Fig. 4a,b ) and incubated the leaves overnight. Then we bombarded the infected leaves with different short DNA oligonucleotides (for example, primer I, Fig. 4b ) and ECFP-expressing plasmid, and left the leaves to incubate for 24 h. DNA oligos can anneal to T-mutRFP-1 in the region where the 1-nt insertion is located ( Fig. 4a,b ). We then used confocal fluorescence microscopy to detect the priming of the DNA oligonucleotides to the T-strand by monitoring the restoration of nuclear RFP expression. EYFP expression was an indicator of successful Agrobacterium -mediated transformation, implying the presence of T-strand T-mutRFP-1 molecules in the EYFP-expressing cells. ECFP expression was used to determine cells in which successful biolistic transformation had occurred, implying that short DNA oligonucleotides had been delivered into those cells. No RFP–NLS-expressing cells were observed in T-mutRFP-1-infected leaves bombarded with only the ECFP plasmid ( Fig. 4c ). RFP–NLS-expressing cells were observed in T-mutRFP-1-infected leaves co-bombarded with ECFP and DNA primer I. The percentage of RFP–NLS-expressing cells in ECFP and EYFP–CHS co-expressing cells was low and we suggest that this can be attributed to the high sensitivity of DNA oligonucleotides to endo- and exonucleases within the transfected cells. We therefore used modified DNA oligonucleotides (that is, primer II, Fig. 4b ) in which several nucleotides were modified with phosphorothioate, which confers higher resistance to nuclease attack. As expected, chemical modification of the DNA oligonucleotides resulted in a higher frequency of RFP–NLS recovery, and 86.1% of the ECFP and EYFP co-expressing cells also expressed RFP–NLS ( Fig. 4c,d ). Next, we produced primer III oligonucleotide which included, in addition to the phosphorothioates, an inverted dT nucleotide at its 3′ end ( Fig. 4b ). This modification is expected to inhibit elongation of the 3′ end of the oligonucleotide by DNA polymerases and by implication, RFP–NLS recovery. Indeed, we observed a lower frequency (59.9%) of RFP–NLS-expressing cells among the ECFP and EYFP co-expressing cells ( Fig. 4c,d ). The difference in RFP–NLS restoration between DNA primer II and primer III was significant ( P <0.01), suggesting that the provided oligonucleotides can act as substrates of the yet-to-be identified plant DNA polymerase(s) in our T-strand-repair assay. The fact that T-strand conversion in T-mutRFP-1-infected and primer III-bombarded cells was less efficient than in their primer II-bombarded counterparts, yet not completely blocked, further indicated involvement of the plant DNA repair machinery in detecting and resolving primer-template mismatch during the process of dsT-DNA formation. 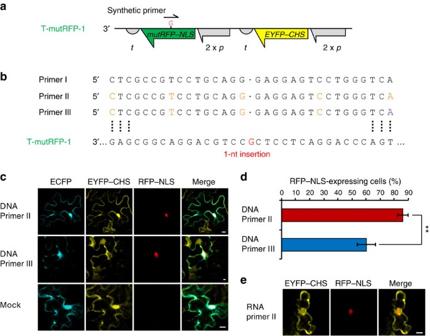Figure 4:In vivopriming of T-strand molecules by synthetic primers. (a) Schematicin vivoannealing of T-mutRFP-1 with synthetic oligonucleotides. (b) Sequences and chemical modifications of DNA primers for biolistic transformation of tobacco. Primers carry wild-type RFP-encoding sequence in the region where T-mutRFP-1 has a 1-nt insertion (red). Orange bases have phosphorothioates modification. Purple base has an inverted dT nucleotide at its 3′ end. (c) Representative images ofAgrobacteriumT-mutRFP-1-infected cells bombarded with a combination of primers and ECFP-expressing plasmid. Scale bars are 10 μm in length. (d) Frequency of RFP–NLS-expressing cells among ECFP and EYFP–CHS co-expressing cells. Data are presented as mean±s.d. (significant difference atP<0.01 in a two-tailedt-test between primer II and primer III assuming unequal variances). (e) Representative images ofAgrobacteriumT-mutRFP-1-infected cells bombarded with an RNA primer sharing the same sequence and chemical modifications as primer II. Scale bars are 10 μm in length. Figure 4: In vivo priming of T-strand molecules by synthetic primers. ( a ) Schematic in vivo annealing of T-mutRFP-1 with synthetic oligonucleotides. ( b ) Sequences and chemical modifications of DNA primers for biolistic transformation of tobacco. Primers carry wild-type RFP-encoding sequence in the region where T-mutRFP-1 has a 1-nt insertion (red). Orange bases have phosphorothioates modification. Purple base has an inverted dT nucleotide at its 3′ end. ( c ) Representative images of Agrobacterium T-mutRFP-1-infected cells bombarded with a combination of primers and ECFP-expressing plasmid. Scale bars are 10 μm in length. ( d ) Frequency of RFP–NLS-expressing cells among ECFP and EYFP–CHS co-expressing cells. Data are presented as mean±s.d. (significant difference at P <0.01 in a two-tailed t -test between primer II and primer III assuming unequal variances). ( e ) Representative images of Agrobacterium T-mutRFP-1-infected cells bombarded with an RNA primer sharing the same sequence and chemical modifications as primer II. Scale bars are 10 μm in length. Full size image We next tested whether RNA primers can also anneal with T-strand molecules and initiate their double-stranded conversion. We bombarded tobacco leaves infected with Agrobacterium as above with RNA primers that had the same sequence and chemical modulation as primer II ( Fig. 4b ). As RNA primers are highly susceptible to contaminating nucleases, we omitted ECFP-expressing plasmid from the bombardment to avoid potential RNA degradation by residual RNase from the plasmid preparation. Confocal fluorescence microscopy analysis of the infected cells revealed that while most of them exhibited only EYFP–CHS expression, 20 individual cells, as shown, for example, in Fig. 4e , also exhibited RFP–NLS expression. No RFP–NLS-expressing cells were detected in leaf samples when an empty bullet was used in the bombardment. Because of the instability of the RNA primer and the extremely low efficiency of putative RNA-mediated DNA repair [28] , we could only detect about 1 or 2 events per leaf sample when using RNA primer II. Whereas, our observations indicated that the RNA primers like DNA primers can also anneal to the incoming T-strand during its conversion to dsT-DNA. Collectively, results of our T-strand-repair assays indicated that T-strand molecules are subjected to DNA repair by the plant machinery, which is active during the conversion to dsT-DNA molecules. Taken together, our data show that T-strand molecules, which are likely to be stripped of their coating proteins before integration [25] , [26] , can interact with DNA and RNA molecules in living cells. Our observations thus suggest a mechanism for T-strand conversion to a dsT-DNA molecule ( Fig. 5 ), in which RNA primers are synthesized de novo in random positions along the T-strand template, and/or endogenous pre-existing ssDNA/RNA fragments randomly anneal to the T-strand. These nucleic acid molecules then serve as primers in the polymerization of the T-DNA nascent strand. Short DNA fragments may derive from DNA fragmentation during the occurrence of genomic DSBs, while RNA primers may be synthesized by primase or derive from various cellular pathways (for example, the plant silencing and DNA polymerization machineries). Such naturally occurring primers may not accurately match the T-strands. It would be interesting to test whether mutations within the T-DNA can indeed arise from natural dsT-DNA formation via incorporation of these putative mismatched DNA/RNA primers, or some unknown mechanism that exists to prevent mutagenesis of T-strand molecules. Interestingly, the reconstruction of RFP–NLS-encoding sequences in mutated T-strands by various type of primers indicates that dsT-DNA molecules are likely subjected to various types of DNA repair by the plant machinery. Our observations thus also provide an alternative, mechanistic explanation for the frequently seen degeneration of the integrated T-DNA molecule’s termini, especially the 3′ end. Combining our results with previously suggested T-DNA integration models [12] , truncation of T-DNA likely occurs during its conversion to double-stranded form, as shown here, and/or during integration, at time when plant DNA processing factors are activated. Studies have shown that two T-DNA molecules deriving from different Agrobacterium cells often integrate at the same genomic location [29] , and that various host proteins may mediate the interaction of T-complexes with plant nucleosomes [7] and aid in stripping T-strands of their coating proteins. It would be intriguing to test whether T-strands can be actively directed to the integration sites where active DNA synthesis and repair are occurring and reagents (that is, DNA or RNA fragments and dNTPs) are abundant for the conversion process. 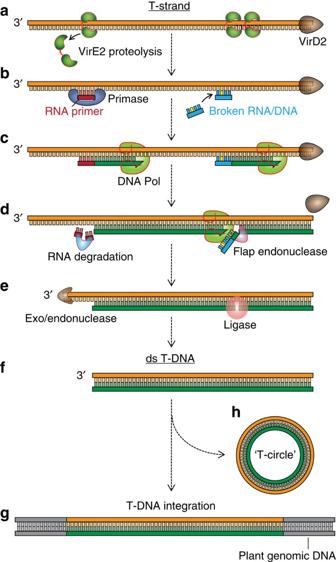Figure 5: Hypothetical model of dsT-DNA formation in plant cells. (a) VirE2 proteins are removed from T-strand molecules by targeted proteolysis. (b) Primase synthesizesde-novoRNA primers using T-strand as the template, and endogenous pre-existing DNA/RNA fragments anneal to the T-strand. Base pair mismatch (shown in yellow) between the primer and the T-strand may lead to mutagenesis in the T-DNA sequence. (c) DNA/RNA primers initiate the nascent strand polymerization, which is carried out by plant DNA polymerase(s). (d) DNA/RNA primer degradation. (e) The unconverted 3′ end of the T-strand is sensitive to nuclease degradation. (f–h) 3′-Truncated dsT-DNA molecules integrate into plant genomic double-strand breaks (g), or ligate intra/inter-molecularly forming the recently identified ‘T-circle’ molecules30(h). Figure 5: Hypothetical model of dsT-DNA formation in plant cells. ( a ) VirE2 proteins are removed from T-strand molecules by targeted proteolysis. ( b ) Primase synthesizes de-novo RNA primers using T-strand as the template, and endogenous pre-existing DNA/RNA fragments anneal to the T-strand. Base pair mismatch (shown in yellow) between the primer and the T-strand may lead to mutagenesis in the T-DNA sequence. ( c ) DNA/RNA primers initiate the nascent strand polymerization, which is carried out by plant DNA polymerase(s). ( d ) DNA/RNA primer degradation. ( e ) The unconverted 3′ end of the T-strand is sensitive to nuclease degradation. ( f – h ) 3′-Truncated dsT-DNA molecules integrate into plant genomic double-strand breaks ( g ), or ligate intra/inter-molecularly forming the recently identified ‘T-circle’ molecules [30] ( h ). Full size image The question remains whether T-strand complementation occurs in close proximity to integration sites and during the integration steps. It was well established that dsT-DNA molecules are potent substrates for genomic integration via DSBs repair [11] , [19] , [20] . It is thus possible that T-strand conversion to dsT-DNA may be, at least in part, a limiting factor in T-DNA integration. Nevertheless, recent evidence suggests that dsT-DNA intermediates can undergo inter/intra-molecular cyclization and form circular molecules that may become incapable for integration [30] . Therefore, dsT-DNA formation and its accessibility to integration may be regulated in a more comprehensive manner. We report here that oligonucleotides can efficiently interact with T-strand molecules in living cells. Thus, while the specific set of proteins involved in the process of T-strand conversion still needs to be identified, our observations suggest a possible strategy to enhance the rate of T-strand conversion to double-stranded form and by implication, to improve the efficiency of gene-replacement and site-specific-integration systems in crops and model plants. DNA constructs We first produced the pSAT1.35S.intGUS.35ST plasmid, in which the intron-containing GUS-encoding sequence (intGUS) was cloned between the dual 35S CaMV promoter and the 35S CaMV terminator, and the entire plant expression cassette was flanked by Asc I sites. We also produced a binary vector, pRCS2-adapter, by replacing the multicloning site of pRCS2 (refs 31 , 32 ) with a single Asc I site. We next transferred the intGUS expression cassette into the Asc I site of the pRCS2-adapter, producing the Agrobacterium ’s binary vectors with sense (S) and antisense (AS) intGUS expression cassettes. We then produced 5′- and 3′-truncated intGUS expression cassettes by PCR on pSAT1.35S.intGUS.35ST template using different primer pairs. S5′: 5′-GGAATTCTGTGCCAGGCAGTTTTAACGA-3′ and 5′-TCCCGAGGGGAACCCTGTGG-3′; AS3′ and AS5′: 5′-AGGCGCGCCTCGTCCACCCAGGTGTT-3′ and 5′-TCCCGAGGGGAACCCTGTGG-3′. The truncated intGUS expression cassettes were next transferred as EcoR I and Asc I (S5′) or Asc I (AS3′ and AS5′) into the same sites of the pRCS2-adapter, producing the Agrobacterium binary vectors S5′, AS3′ and AS5′. The T-RFP binary vector was constructed by cloning the EYFP–CHS (that is, yellow fluorescent protein (EYFP) tagged with ER-bound CHS) and the RFP–NLS (that is, the RFP tagged with a NLS) expression cassettes [31] into a single binary vector. More specifically, the EYFP–CHS and RFP–NLS expression cassettes driven by dual 35S promoter were subsequently cloned as PI- Psp I and I- Ceu I fragments into the I- Ceu I and I- Sce I sites of pRCS2 (refs 31 , 32 ), respectively. To construct T-mutRFP-1 and T-mutRFP-2, we first performed PCR on T-RFP template using primers with extra 1 or 11 nt. T-mutRFP-1: 5′-AACTGCAGGCGAGGAGTCCTGGGTCACGGTCACCA-3′ and 5′-AACTGCAGGCATCTTGGCTATTGGCACT-3′; T-mutRFP-2: 5′-AACTGCAGGAACCAATTCATGAGGAGTCCTGGGTCACGGTCACCA-3′ and 5′-AACTGCAGGCATCTTGGCTATTGGCACT-3′. The PstI-digested PCR products were then cloned into the Sbf I sites of the T-RFP plasmid, replacing the wild-type RFP-coding sequence. To produce cRFP and anti-cRFP, a small portion of the wild-type RFP CDS was amplified by PCR using different primer pairs. cRFP: 5′-GGCGCGCCCTTGGCCATGTAGGTGGTCT-3′ and 5′-GGAATTCCGAGGACGTCATCAAGGAGT-3′; anti-cRFP: 5′-GGCGCGCCCTTGGCCATGTAGGTGGTCT-3′ and 5′-GGCGCGCCCGAGGACGTCATCAAGGAGT-3′. PCR fragments were then transferred as EcoR I and Asc I (cRFP) or Asc I (anti-cRFP) into the same sites of the pRCS2-adapter. mut-RFP was produced by PstI digestion, Klenow overhang removal and re-ligation of cRFP. pSAT6.35SP.ECFP-C1.35ST, in which a ECFP-encoding sequence was cloned between the dual 35S CaMV promoter and the 35S CaMV terminator, was used to monitor biolistic transfection efficiency [32] . Transient expression Binary vectors were transferred into A. tumefaciens strain EHA105. For the T-DNA repair assay, Agrobacterium cells were grown overnight at 28 °C in YEP medium supplemented with 80 μg ml −1 spectinomycin and 200 μg ml −1 streptomycin, collected by centrifugation for 10 min at 3,000 g and resuspended in induction medium (10.5 g l −1 K 2 HPO 4 , 4.5 g l −1 KH 2 PO 4 , 1 g l −1 (NH 4 ) 2 HPO 4 , 0.5 g l −1 sodium citrate, 1 g l −1 glucose, 1 g l −1 fructose, 4 g l −1 glycerol, 120 mg l −1 MgSO 4 , 2 g l −1 2-( N -morpholine)-ethanesulphonic acid, pH 5.6) supplemented with 100 μM acetosyringone and antibiotics. They were then grown to an OD 600 of 0.6, again collected by centrifugation for 10 min at 3,000 g and resuspended in infiltration medium (10 mM MgSO 4 ,10 mM 2-( N -morpholine)-ethanesulphonic acid, pH 5.6) supplemented with 200 μM acetosyringone to an OD 600 of 0.2. The Agrobacterium infiltration of N. tabacum adopted protocol reported by Van der Hoorn et al . [33] More specifically, Agrobacterium cultures were infiltrated using a 2-ml sterile syringe into fresh leaves of 4- to 5-week-old tobacco plants. Bacterial cultures used in all infiltration experiments within the same panel in Fig. 1 had the same cell concentration. Cell-number ratio of Agrobacterium was 1:1 between T-RFP and T-mutRFP-1 and 1:9 between T-mutRFP-1 and cRFP/anti-cRFP, shown in Fig. 3 . Tobacco explants were collected at the specified time or 48 h (if not specified) after infiltration. Explants were then subjected to GUS-staining analysis or confocal fluorescence microscopy. GUS-staining analysis was performed according to Jefferson et al . [34] More specially, infected explants were vacuum infiltrated with the chromatogenic substrate X-Gluc and incubated at 37 °C overnight. Explants were then de-stained with 70% ethanol at room temperature for several days. Molecular analysis of infected plants Total plant DNA was extracted from leaves of infected tobacco 48 h after Agrobacterium infiltration using the phenol-chloroform method. The region surrounding T-RFP and mut-cRFP hybridization was amplified by PCR using primers 5′-CCAGCTTGATGTCGGTCT-3′ and 5′-GATAGCCATGGCCTCCT-3′. The resulting PCR fragment was digested with PstI for 4 h. DNA digestion was visualized by standard agarose gel electrophoresis. Biolistic transfection Biolistic transfection was carried out using the Bio-Rad Helios Gene Gun System as instructed by the manufacturer ( http://www.bio-rad.com ). The transfection control plasmid pSAT6.35SP.ECFP-C1.35ST was prepared using the Qiagen Plasmid MidiPrep Kit. DNA and RNA oligonucleotides used in the biolistic transfection were purchased from IDT (Coralville, IA). Plasmid (5 μg) and oligonucleotides (25 μg) were fully mixed before precipitation on the gold bullets. Fresh leaves from 4- to 5-week-old tobacco plants were used in this experiment. Confocal microscopy Plant tissue was viewed directly with a confocal laser scanning microscope (TCS SP5; Leica). EYFP was excited with an argon laser at 514 nm, and fluorescence was monitored between 520 and 542 nm. RFP was excited with a helium-neon laser at 561 nm, and fluorescence was monitored between 607 and 642 nm. ECFP was excited with an argon laser at 458 nm, and fluorescence was monitored between 465 and 514 nm. Chlorophyll fluorescence was monitored above 700 nm. Sequential scanning was implemented to detect different fluorescence. How to cite this article: Liang, Z. and Tzfira, T. In vivo formation of double-stranded T-DNA molecules by T-strand priming. Nat. Commun. 4:2253 doi: 10.1038/ncomms3253 (2013).